Biomimetic superelastic graphene-based cellular monoliths Many applications proposed for graphene require multiple sheets be assembled into a monolithic structure. The ability to maintain structural integrity upon large deformation is essential to ensure a macroscopic material which functions reliably. However, it has remained a great challenge to achieve high elasticity in three-dimensional graphene networks. Here we report that the marriage of graphene chemistry with ice physics can lead to the formation of ultralight and superelastic graphene-based cellular monoliths. Mimicking the hierarchical structure of natural cork, the resulting materials can sustain their structural integrity under a load of >50,000 times their own weight and can rapidly recover from >80% compression. The unique biomimetic hierarchical structure also provides this new class of elastomers with exceptionally high energy absorption capability and good electrical conductivity. The successful synthesis of such fascinating materials paves the way to explore the application of graphene in a self-supporting, structurally adaptive and 3D macroscopic form. Graphene, combining extraordinary mechanical, electrical and thermal properties as well as ease of scalable synthesis from inexpensive graphite, holds great promise as an exceptional nansocale building block for constructing macroscopic three-dimensional (3D) bulk assemblies for widespread applications [1] , [2] , [3] , [4] . A number of methods, such as self-gelation and chemical vapour deposition (CVD) over a porous catalyst have recently been developed to fabricate highly porous graphene cellular monoliths [5] , [6] , [7] , [8] , [9] , [10] , [11] , [12] . However, as with most of the existing porous carbon materials [13] , the resulting graphene monoliths are generally brittle and have small recoverable deformation before failure unless they are infiltrated with an elastomeric polymer [5] or grown on pre-formed carbon nanotube aerogels [14] . Superelasticity that has been observed in foams made of carbon-based tubular or fibrillar nanostructures [15] , [16] , [17] , [18] , [19] , [20] , [21] has not been achieved in foams solely based on graphene sheets. Indeed, as the specific elastic bending stiffness of a sheet-like structure is known to be intrinsically inferior to that of its tubular or fibrillar counterparts [22] , previous analysis [13] suggests that it would be highly challenging to realize superelasticity in graphene foams. The ability to maintain structural integrity upon large deformation for graphene monoliths is not only crucial for building new types of flexible electronic devices, such as batteries, supercapacitors, sensors and actuators, but also important for future development of carbon-based biological tissue scaffolds and ultralight cellular materials for mechanical damping and thermal/acoustic insulation. It is thus highly desirable to develop new strategies to tackle this challenging but very important problem. The properties of cellular solids are dictated by the intrinsic properties of the solid phase, the density and the cell geometry [23] , [24] . To design an appropriate structure that can allow the extraordinary mechanical properties of individual graphene sheets to be harnessed in a monolithic structure effectively, we examined a variety of existing cellular materials [23] , [25] and were particularly impressed by the high mechanical efficiency of natural cork’s hierarchical structure. Cork is one of the oldest natural materials exploited and used by human beings [23] . Modern structural analysis has revealed how nature makes biological cellular materials lightweight yet mechanically resilient. In wood and cork, cellulose nanofibers in the cell walls are closely packed in a highly ordered manner to maximize strength [26] . Individual cells with a dimension of tens of micrometres are then intimately connected to form a honeycomb-like structure [23] , [25] , a geometry that has proven to be highly beneficial to maximize bulk-specific elastic modulus [23] , [27] . Efficient assembly at all the structural levels is the key for lightweight cork to achieve high specific mechanical strength and elasticity. We thus surmised that graphene monoliths could deliver striking mechanical properties if they could be hierarchically structured in a similar manner as cork. In the present work, we demonstrate that graphene monoliths with a cork-like hierarchical structure can be readily fabricated by freeze casting of partially reduced graphene oxide (GO). The resulting biomimetic graphene-based monoliths exhibit a combination of ultralow density, superelasticity, good electrical conductivity and high efficiency of energy absorption. Formation cork-like graphene monoliths via freeze casting We explored a versatile, readily accessible and inexpensive solution-phase materials shaping technique, namely freeze casting, to explore the possibility of assembling graphene sheets into cork-like monoliths. Previous studies have demonstrated that when an aqueous suspension of nanoparticles is frozen, phase separation can result in the rejection of solid nanoparticles from the forming ice, which are then accumulated between the growing ice crystals [28] , [29] . If the fraction of nanoparticles is higher than the percolation threshold, the entrapped particles can form a continuous 3D network. Subsequent sublimation of ice results in the formation of a porous solid material. Freeze casting has been successfully adopted to synthesize a variety of porous ceramic, metallic, polymeric and composite materials, including carbon nanotubes or graphene-based polymer composites [18] , [30] , [31] , [32] , [33] . Although previous research on freeze casting has been centred on polymers and spherical particles [28] , [29] , we were particularly interested in studying how 2D graphene sheets interact with anisotropic ice crystal growth without the interference of other polymer or surfactant additives. In this work, GO, which can be readily produced from graphite in large quantities [2] , was chosen as a precursor to synthesize graphene-based monoliths. The porous structure resulted from the freeze-casting method is governed by complex and dynamic liquid–particle and particle–particle interactions [28] . We found that the amount of oxygen-containing groups of GO has a significant effect on such interactions. Consequently, the structure of the resulting materials is strongly related to the chemistry of GO ( Supplementary Methods , Supplementary Figs S1 and S2 ). Water-soluble GO appears to be the ideal precursor for freeze casting. However, we found that directly freezing of GO dispersions only resulted in a randomly oriented porous structure, which is consistent with a previous report [34] . The monoliths directly resulted from unreduced GO displayed poor mechanical strength and small recoverable deformation region ( Supplementary Methods ). By carefully controlling both the amount of oxygen-containing groups of GO (simply via reduction time) and freezing conditions (see details in Supplementary Methods ), we found that a cork-like graphene cellular structure could be readily obtained when the carbon/oxygen atomic ratio in partially reduced GO (denoted as pr-GO) was tuned to be around 1.93 (see Supplementary Table S1 ). Of particular interest is that freezing also simultaneously induced the pr-GO sheets in each cell wall to be organized in a highly ordered fashion, mimicking the manner of cork’s structuring on both the nanometre and micrometre scales. 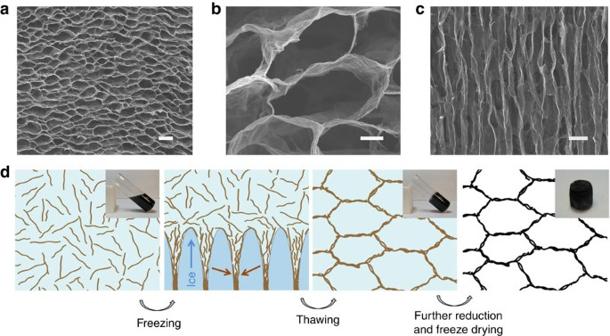Figure 1 Morphology and formation mechanism of the cork-like graphene elastomer. (a–c) Typical top-view (a,b) and side-view (c) SEM images of graphene monolith of 5.10 mg cm−3. (d) Schematic showing the formation mechanism of the cork-like monolith by freeze casting. When a well-dispersed pr-GO dispersion (the first scheme) is frozen, pr-GO sheets are concentrated at the boundary of ice crystals and then aligned along the growth direction of ice due to the squeezing effect (the second scheme, side-view). As a result, a continuous honeycomb-like network is formed. The network retains its connectivity when the ice is thawed (the third scheme, top-view). The pr-GO sheets are illustrated as slightly corrugated lines in the scheme with the brown representing partially reduced, whereas the black for fully reduced. Photos of the corresponding samples are presented in the insets. Scale bars, 50 μm (a,c) and 10 μm (b). Figure 1a–c presents typical scanning electron microscope (SEM) images of an as-formed graphene-based monolith with a density of 5.10 mg cm −3 . The sample was prepared by freezing an aqueous solution of pr-GO in a dry ice bath, followed by thawing, further reduction, freeze drying and annealing at 200 °C. Resembling cork [23] , [25] , the monolith exhibits a honeycomb-like cellular structure with the cell dimension in the order of tens of micrometres and the cell walls slightly corrugated, despite the thickness of the cell wall being ~100 times thinner than that of the cork (~1 μm) (ref.23 [23] ). High-resolution transmission electron microscopy (HRTEM) analysis ( Fig. 2a ) revealed that the graphene sheets in the cell wall are well oriented in a nearly parallel manner, similar to the layered structure observed in the ultrastrong graphene paper prepared under the directional flow [35] , [36] . Figure 1 Morphology and formation mechanism of the cork-like graphene elastomer . ( a – c ) Typical top-view ( a , b ) and side-view ( c ) SEM images of graphene monolith of 5.10 mg cm −3 . ( d ) Schematic showing the formation mechanism of the cork-like monolith by freeze casting. When a well-dispersed pr-GO dispersion (the first scheme) is frozen, pr-GO sheets are concentrated at the boundary of ice crystals and then aligned along the growth direction of ice due to the squeezing effect (the second scheme, side-view). As a result, a continuous honeycomb-like network is formed. The network retains its connectivity when the ice is thawed (the third scheme, top-view). The pr-GO sheets are illustrated as slightly corrugated lines in the scheme with the brown representing partially reduced, whereas the black for fully reduced. Photos of the corresponding samples are presented in the insets. Scale bars, 50 μm ( a , c ) and 10 μm ( b ). 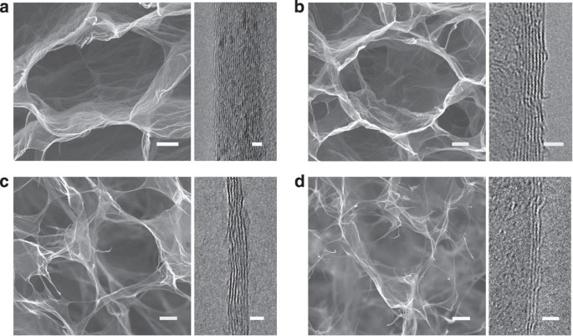Figure 2 Morphology and structure of the graphene elastomers with different densities. (a–d) SEM (left) and TEM (right) images of monoliths with a density of 5.10 (a), 2.65 (b), 1.10 (c) and 0.56 mg cm−3(d). Scale bars are 10 μm in all SEM images and 2 nm in all TEM images. Full size image Figure 2 Morphology and structure of the graphene elastomers with different densities . ( a – d ) SEM (left) and TEM (right) images of monoliths with a density of 5.10 ( a ), 2.65 ( b ), 1.10 ( c ) and 0.56 mg cm −3 ( d ). Scale bars are 10 μm in all SEM images and 2 nm in all TEM images. Full size image In conjunction with the anisotropic structure of GO, the principle of the freeze-casting process that has previously been proposed for other nanoparticle suspensions [30] , [31] can be extended to elucidate the formation of such a unique cellular structure. As schematically illustrated in Fig. 1d , upon freezing, the partially reduced GO sheets are rejected from the forming ice and entrapped between neighbouring ice crystals to form a continuous network whose structure is determined by ice crystal template. As the growth rate of ice crystals is highly anisotropic (varied by 2–3 orders of magnitude along different growing directions [28] , [29] ), the 2D pr-GO sheets are forced to align along the moving solidification front, while they are concentrated and then squeezed at the crystal boundaries, yielding a highly ordered layered assembly. Furthermore, because the π–π attraction between pr-GO sheets is enhanced as a result of partial reduction, the as-formed network was found to be quite stable and could maintain its structural integrity upon thawing. This allowed us to perform an additional step to maximally reduce GO in solution and further increase the intersheet π–π attraction. Once the network was strengthened by such treatments, further freezing was found to have little effect on the structure of network. Characterization of mechanical properties Compression tests revealed that the as-formed graphene monolith exhibited excellent resilience when released from compression. Similar to cork and other elastomeric foams [23] , three regimes of deformation can be observed in the loading stress–strain curve: nearly linear elastic regime, corresponding to bending of the cell walls; relatively flat stress plateau, corresponding to elastic buckling of cell walls; and abrupt stress increasing regime, corresponding to densification of cells ( Fig. 3a ). For the first compression cycle, the nearly linear elastic region of the graphene monolith extends up to ~20% strain, much higher than that of other polymeric foams (~up to 10%) [23] . The compressive stress is ~8 kPa at the plateau, and is 18 kPa at 80% strain for the monolith with density of 5.10 mg cm −3 . These compressive stress values are 2–9 times higher than those of other carbon-based foams with a similar or twice the density [18] , [19] and are comparable to that of metallic lattice [24] with a density of 14 mg cm −3 . At 80% strain, the graphene monolith can support over 50,000 times of its own weight without collapsing, which has rarely been found in other foam-like materials. 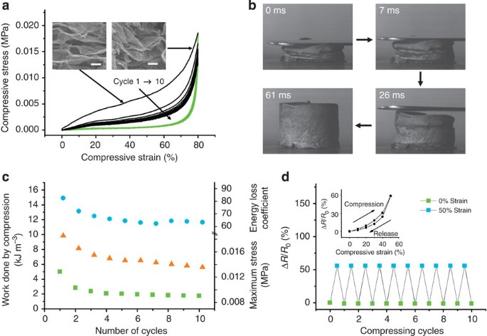Figure 3 Multicycle compressive properties of the graphene elastomer with a density of 5.10 mg cm−3. (a) Compressive stress–strain curves of 10 cycles of loading (black lines) and unloading (green lines). The inserts show the SEM images of elastomer under compression at different strains. Scale bars, 10 μm. (b) A set of real-time images of a compressed sample showing the recovering process. (c) Work done by compression (green squares), maximum stress at 80% strain (orange triangles) and energy loss coefficient (blue circles) during the first 10 compression cycles (calculated from the stress–strain curves shown in panela). (d) Electrical resistance change when repeatedly compressed up to 50% of strain for over 10 cycles. The insert shows the result for one cycle. Scale bars, 10 μm (a). Figure 3 Multicycle compressive properties of the graphene elastomer with a density of 5.10 mg cm −3 . ( a ) Compressive stress–strain curves of 10 cycles of loading (black lines) and unloading (green lines). The inserts show the SEM images of elastomer under compression at different strains. Scale bars, 10 μm. ( b ) A set of real-time images of a compressed sample showing the recovering process. ( c ) Work done by compression (green squares), maximum stress at 80% strain (orange triangles) and energy loss coefficient (blue circles) during the first 10 compression cycles (calculated from the stress–strain curves shown in panel a ). ( d ) Electrical resistance change when repeatedly compressed up to 50% of strain for over 10 cycles. The insert shows the result for one cycle. Scale bars, 10 μm ( a ). Full size image More interestingly, the graphene monolith could be compressed to at least 80% strain and was still able to almost completely recover to its original shape rapidly when the loading was removed. As shown in Fig. 3b and Supplementary Movie 1 , the compressed monolith can bounce back to its original size at the speed of >7,000 mm min −1 . The highly elastic graphene monolith also exhibited excellent cycling performance. No significant decrease in terms of work done by compression, maximum stress at 80% strain as well as energy loss coefficient was observed after four cycles of compressive loading and unloading ( Fig. 3c ). After being compressed for 1,000 cycles, the graphene monolith only experienced 7% reduction in thickness and still retained over 76% of maximum stress ( Supplementary Fig. S4 ). Additionally, the response of bulk electrical resistance of the monolith is also highly constant over multiple cycles of compression ( Fig. 3d ), further indicating its remarkable structural resilience. The exceptional elasticity observed in our graphene monolith was a surprise to us. According to the literature [13] , all the existing carbon foams and porous carbons except for those made of fibrous carbon [15] , [17] , [19] , [21] or graphitic ribbons [20] are prone to failure in a brittle manner when subjected to macroscopic deformation. Previous studies suggest that when foam made of mono- or very few layers of graphene is severely compressed, the intersheet van der Waals adhesion would overwhelm the elastic energy stored, preventing elastic recovery [13] , [37] . Indeed, superelasticity has not been observed in randomly structured graphene foams or aerogels prepared by CVD [5] or self-gelation [6] , [7] , [9] , [11] . We also found that graphene foams with a poorly organized structure and much smaller cell sizes prepared from the same GO precursor all collapsed when subjected to severe compression ( Supplementary Fig. S3 ). We thus believe that it is the unique cork-like hierarchical structure of our graphene monolith that has enabled the unusual high elasticity and mechanical robustness. On the top level, the cells are organized in a honeycomb-like manner to maximize the elastic modulus and strength. On the lower level, the cell wall is comprised of multilayers of face-to-face oriented graphene sheets. As observed in layered GO paper [35] , the formation of such an ordered, tightly packed multilayered structure can maximize the π–π interactions between layers and thus greatly enhance its strength and elastic stiffness (bending stiffness of a film being proportional to cubic of thickness [23] ), allowing the van der Waals adhesion to be overcome by the elastic energy. Meanwhile, the tightly packed cell wall has a thickness of only ~10 nm, rendering a high compliance in the out-of-plane direction and a capability to accommodate a severe bending deformation. Additionally, the corrugation of the cell walls can further enhance the elastic bending stiffness and retard the van der Waals adhesion [38] . The advantages of having a mechanically efficient, biomimetic hierarchical structure can be further demonstrated by our successful synthesis of such monoliths at lower densities with no requirement for any additional polymer binders. We have obtained graphene monoliths with varied densities simply by adjusting the concentration of the starting GO dispersion and their mechanical properties are presented in Supplementary Figs S5 and S6 and Supplementary Table S2 . Thanks to the well-organized hierarchical structure, their compressive modulus E was found to scale with density ρ as E ~ ρ 2 ( Fig. 4a ), indicating the highly efficient structure of graphene monoliths. This relationship is consistent with those observed in other highly efficient cellular materials [23] and nickel metallic lattice [24] . In contrast, most of the existing porous carbon materials generally follow E ~ ρ 3 ( Fig. 4a ) [21] , [39] . As revealed by the SEM and TEM ( Fig. 2 ) as well as electron diffraction analysis ( Supplementary Fig. S7 ), the number of stacked graphene sheets in the cell wall decreases with lowering the density. The lowest density of graphene elastomer we have obtained is ~0.5 mg cm −3 , corresponding to a porosity of 99.98%. This density is nearly four times lower than that of the most lightweight CVD-grown graphene foams (≥2 mg cm −3 ) ( [5] ) and is approximately half of that of ultralight nickel lattice recently reported (≥0.9 mg cm − 3 ) ( [24] ). Noteworthy is that fibrous structures started to appear when the density was reduced to lower than 1.1 mg cm −3 ( Fig. 2 ). HRTEM analysis revealed that they were the result of scrolling of graphene sheets ( Supplementary Fig. S8 ). This is in agreement with the theoretical prediction that a free-standing ultrathin graphene sheet is prone to rolling up to form a tubular structure [40] . Scrolling of a sheet-like material is known to enhance the elastic stiffness remarkably [22] . Thus, the fibrous structure resulted from self scrolling of single or few layers of graphene helps maintain elasticity and structural integrity as well when the density of the graphene monolith becomes extremely low. 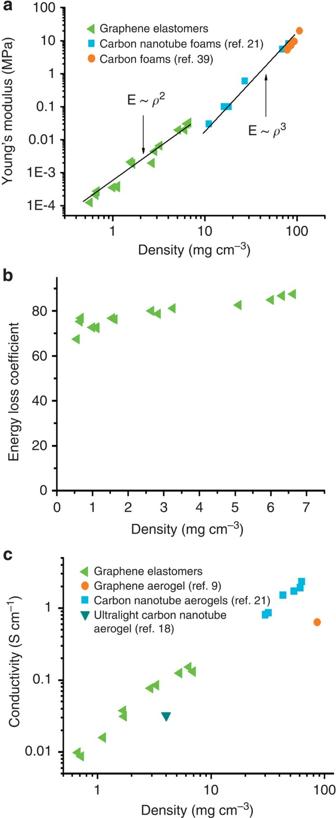Figure 4:Physical properties of graphene elastomers with different densities. The data for selected low-density porous carbon materials are also presented for comparison. (a) The relationship between Young’s modulus and density of graphene elastomers. (b) The energy loss coefficient (the ratio of dissipated energy over total work done during the compression). (c) Electrical conductivity of graphene elastomers. Figure 4: Physical properties of graphene elastomers with different densities. The data for selected low-density porous carbon materials are also presented for comparison. ( a ) The relationship between Young’s modulus and density of graphene elastomers. ( b ) The energy loss coefficient (the ratio of dissipated energy over total work done during the compression). ( c ) Electrical conductivity of graphene elastomers. Full size image Energy absorption capability and electrical conductivity Energy absorption or dissipation is one of the key functions of cellular foams [23] . Our graphene elastomers exhibit excellent energy absorption capability. Depending on the density, the energy loss coefficient of graphene elastomers ranges from 67 to 87% ( Fig. 4b ), which is much higher than that of conventional carbon, metallic and polymer foams [15] , [24] , [41] . For example, the sample with a density of 5.10 mg cm −3 gives an energy loss coefficient of 82.5% at the first compressive cycle and ~65% after four cycles of compression ( Fig. 3c ), in comparison to 77% (first cycle) and 40% (after three cycles) for the metallic micro-lattice [24] , 65% for the first compression cycle of dense carbon nanotube foam [15] . To our knowledge, no other foams could offer such high-energy loss coefficients and fast elastic recovery simultaneously. In terms of the energy dissipation mechanism, the excellent cycling performance of the elastomers rules out the possibility of fracture and friction between broken fragments of cell walls, as is often observed in other cellular materials such as metallic lattice [24] . The effect of compression of air is negligible because of the open-cell structure of the graphene elastomers and the low stain rate (≤3,000% per min) used in our experiments. The compression experiments at different strain rates (10–3,000% per minute) revealed that the stress–strain curve was almost independent on the strain rate. Similar to other dense carbon viscoelastic materials [16] , [42] , the high-energy loss coefficient could be attributed to the intersheet van der Waals adhesion and frictions during bending/buckling in the compression and the unloading process, as well as de-binding of the contacted cell walls when unloaded. The face-to-face oriented stacking configuration of graphene sheets in the cell wall maximizes the contact area between graphene sheets, which can generate frictions that are comparable to or even higher than that of dense carbon nanotube structures [15] . The increase in energy loss coefficient with density of the elastomer appears to support the above speculation ( Fig. 4b ). The unique hierarchical structure of graphene elastomers also gives rise to high electrical conductivity. The high level of sheet–sheet connectivity and self-orientation of graphene sheets ensures an excellent electrical conduction path in the monoliths. Indeed, the electrical conductivity of the graphene elastomer with a density of 5.10 mg cm −3 was measured to be 0.12 S cm −1 ( Fig. 4c ), three times higher than that of carbon nanotube aerogel with a similar density [18] . The combination of high aspect ratio and 2D structure of inherently stiff graphene sheets, face-to-face oriented stacking configuration in the cell wall and the honeycomb-like cell structure has made all these exceptional mechanical and electrical properties possible. In conclusion, we have demonstrated that ultralight graphene-based cellular monoliths can be made superelastic by mimicking the hierarchical structure of cork through a cost-effective freeze-casting process. With ultralow density, superelasticity with an extremely high recovery rate, good electrical conductivity, high efficiency of energy absorption and ease of synthesis all combined together, we anticipate that such exceptional carbon-based cellular materials will open up numerous opportunities for a range of technological areas. In particular, our discovery makes it possible to explore the properties and applications of graphene in a self-supporting, structurally adaptive and 3D macroscopic form. This work will thus pave the way for new types of graphene-based flexible devices. Furthermore, other functional materials can be readily incorporated into the open void space, offering plenty of room to fabricate many new graphene-based nanocomposites. Preparation of elastomeric graphene monoliths GO aqueous dispersions were prepared using a similar method, we previously reported except that graphite oxide was dispersed using a bath sonicator (Branson, B2500R) [43] . The lateral size of the resulting of GO sheets ranged from 0.2 to 10 μm. In a typical procedure for synthesis of a graphene monolith of 5.10 mg cm −3 , GO solution (1.5 ml, 5 mg ml −1 ) was mixed with ascorbic acid (15 mg) in a 4-ml cylindrical glass vial, which was then placed in boiling water bath for 30 min to obtain a partially reduced GO dispersion. The vial was then immersed in a dry ice bath to freeze for 0.5 h. After being thawed at room temperature, the vial was placed in a boiling water bath to further reduce GO for 8 h. The obtained gel was then sequentially subjected to dialysis in water (to remove soluble species), freezing drying and thermal annealing at 200 °C in air for 2 h. Graphene monoliths with a range of density (from 0.5 to 6.6 mg cm −3 ) were prepared under the same conditions except using different concentrations of GO (0.5–7.0 mg ml −1 ) and the ratio of GO to ascorbic acid by weight was kept consistent at 1:2. Note that synthesis of graphene monoliths with a density higher than 6.6 mg cm −3 appear to be difficult as it is challenging to obtain a well-dispersed GO dispersion with a concentration higher than 7.0 mg ml −1 . Characterization The dimensions and weight of elastomers were determined with a caliper (Stamvick) with an accuracy of 0.01 mm and a balance (AND GH-252) with an accuracy of 0.01 mg. Following the standard practice in the field of cellular materials [24] , the density of the monoliths was calculated by the weight of the solid content without including the weight of air entrapped (as the samples were weighted in air, the weight of air was automatically extracted). The SEM and TEM images were obtained using a JOEL 7001F SEM and an aberration-corrected TEM (FEI Company) operated at 80 kV, respectively. The samples were prepared in cylindrical shape (~12 mm in diameter and 8 mm in height) for compressive tests and electrical conductivity measurements. The compressive tests were performed in an Instron (Micro Tester, 5848, Instron) using a 10 N load cell and strain control mode with a strain rate of 100% per minute. Filming of the recovery of a compressed graphene monolith was recorded using a high-speed camera operated at 700 frames per second. The electrical conductivity was determined by a two-probe method. To optimize the electrical contact between copper wires and elastomer, both ends of elastomer were carefully coated with a thin layer of silver paste. The monitoring of electrical resistance in relation to the number of mechanical compression was performed under a laser displacement sensor (LK-GD500, Keyence) and the change of electrical resistance was measured by a potentiostat (Model 363, Princeton Applied Research) controlled by an electronic digital interface (e-corder 401, eDAQ) with E-chart data acquisition programme (E-chart, eDAQ). How to cite this article: Qiu, L. et al . Biomimetic superelastic graphene-based cellular monoliths. Nat. Commun. 3:1241 doi: 10.1038/ncomms2251 (2012).